The genetic prehistory of southern Africa Southern and eastern African populations that speak non-Bantu languages with click consonants are known to harbour some of the most ancient genetic lineages in humans, but their relationships are poorly understood. Here, we report data from 23 populations analysed at over half a million single-nucleotide polymorphisms, using a genome-wide array designed for studying human history. The southern African Khoisan fall into two genetic groups, loosely corresponding to the northwestern and southeastern Kalahari, which we show separated within the last 30,000 years. We find that all individuals derive at least a few percent of their genomes from admixture with non-Khoisan populations that began ∼ 1,200 years ago. In addition, the East African Hadza and Sandawe derive a fraction of their ancestry from admixture with a population related to the Khoisan, supporting the hypothesis of an ancient link between southern and eastern Africa. The prehistory of the populations of southern Africa who speak non-Bantu languages with click consonants (hereafter referred to as Khoisan without implying linguistic unity) is poorly understood. A major open question concerns the relationships among these populations, who harbour extensive linguistic diversity (there are three Khoisan language families [1] , [2] , [3] , [4] ) as well as variable modes of subsistence (while most Khoisan groups are hunter-gatherers, some are pastoralists). A second major question concerns the historical relationships of the southern African populations to two populations in eastern Africa who are or previously were hunter-gatherers and who also speak languages with click consonants (the Hadza and Sandawe). It has been hypothesized that the eastern Africans descend, in part, from a Khoisan-related hunter-gatherer population that once occupied a region ranging over much of southern and eastern Africa [5] . However, the anthropological and archaeological evidence for this hypothesis is contested [6] , [7] . Apart from the shared use of click consonants, there is no linguistic evidence that the non-Bantu languages in southern Africa and Hadza stem from a common ancestor [8] , [9] , [10] , although a potential ancestral link between Sandawe and the Khoe-Kwadi family has been suggested [4] , [11] . Genomic studies have the potential to shed new light on the history of the Khoisan. Previous genetic studies based largely on single loci (mitochondrial DNA and the Y chromosome) have documented that the Khoisan carry some of the most ancient lineages in humans [12] , [13] and have suggested deep genetic links between the Khoisan and the Sandawe and Hadza [13] . However, single-locus studies have limited resolution. Although some genome-wide studies have included southern Africans, they have largely focused on a single Khoisan group, making it impossible to elucidate relationships among these populations [14] , [15] , [16] . The few studies of more than one Khoisan group have not included enough populations to form a clear picture of the pattern of sub-structure and population relationships within southern Africa [17] , [18] . Here we present a high-resolution study of the genomic relationships of southern and eastern African populations who speak languages characterized by heavy use of click consonants. Our study capitalizes on three novel resources: (1) a unique collection of southern African DNA samples encompassing most of the linguistic and cultural diversity of Khoisan groups; (2) a single nucleotide polymorphism (SNP) array that is the first to include polymorphisms discovered in Khoisan; and (3) new methods of statistical analysis, some of which we introduce here for the first time, that allow us to make inferences about historical relationships even in the presence of admixture. Data set We genotyped 565,259 SNPs in 187 individuals from 22 African populations (16 Khoisan populations and 5 neighbouring populations speaking Bantu languages shown in Fig. 1a , plus the Hadza) using the Affymetrix Human Origins array [19] . This array is specifically designed for studies of population history: it contains panels of SNPs discovered by sequencing a single individual of known ancestry (including a Khoisan individual), providing precise control of the SNP ascertainment scheme and making it possible to answer questions that are more difficult to address using data from SNP arrays designed for medical genetics. We genotyped populations speaking languages from all three Khoisan language families (Tuu, Kx'a and Khoe-Kwadi [1] , [2] , [3] , [4] , [8] ; Supplementary Table S1 , Supplementary Fig. S1 ). We then merged the data with whole-genome sequencing data from five Sandawe individuals and four Hadza individuals [20] . Finally, we supplemented this with previously collected Affymetrix Human Origins array data on Dinka, Mbuti, Biaka, Yoruba and other African and non-African populations [19] , [21] . 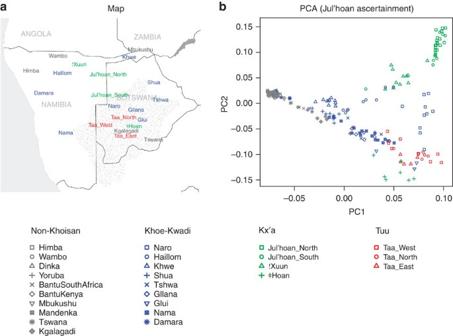Figure 1: Population structure in southern Africa. (a) Approximate locations of sampled populations. Populations are coloured according to linguistic affiliation, as indicated in the legend andSupplementary Fig. S1. The speckled region is the Kalahari semi-desert. (b) PCA on SNPs ascertained in a Ju|'hoan individual. Shown are the positions of each individual along the first and second axes of genetic variation, with symbols denoting the individual's population and linguistic affiliation using the same colour coding as in panela. Figure 1: Population structure in southern Africa. ( a ) Approximate locations of sampled populations. Populations are coloured according to linguistic affiliation, as indicated in the legend and Supplementary Fig. S1 . The speckled region is the Kalahari semi-desert. ( b ) PCA on SNPs ascertained in a Ju|'hoan individual. Shown are the positions of each individual along the first and second axes of genetic variation, with symbols denoting the individual's population and linguistic affiliation using the same colour coding as in panel a . Full size image The Khoisan genetically cluster into two major groups We performed a qualitative exploration of southern African population relationships using principal component analysis (PCA; [22] Supplementary Figs S2–S5 ). We capitalized on the design of the Human Origins array by performing the analysis using three different panels of SNPs, each of which reveals different aspects of population structure ( Supplementary Fig. S4 ). The Yoruba SNPs highlight structure within non-Khoisan Africans, whereas the French SNPs highlight European ancestry in the Nama (consistent with historic documentation [23] ) and hint at European or East African ancestry in some Khoe groups ( Supplementary Figs S4, S6 ). The SNPs ascertained in a Ju|'hoan individual (HGDP 'San') reveal structure invisible to the other panels ( Fig. 1b ). The PCA based on these SNPs divides Africans into three broad clusters: a predominantly non-Khoisan cluster and two Khoisan clusters. The Khoisan clusters do not correspond to linguistic affiliation; whereas one is comprised of Ju|'hoan_North and Ju|'hoan_South, who speak closely related languages/dialects, the other includes populations speaking languages belonging to all three language families ( Supplementary Fig. S1 ). The Khoisan clusters instead reflect geography, corresponding roughly to the northwestern (NW) and southeastern (SE) Kalahari ( Fig. 1a ). On a fine scale, the PCA plot also identifies sub-structure within individual populations ( Supplementary Methods ), as well as cases of discordance between linguistic and genetic affiliation that suggest language shift with little accompanying gene flow. A particularly striking example is the Damara, who cluster with non-Khoisan populations despite speaking a Khoe language. This suggests that the Damara were a non-Khoisan population who acquired their language from their Khoisan neighbours (the Nama [24] ) with little Khoisan gene flow [25] . Admixture in southern Africa related to the Bantu expansion A number of populations occupy intermediate positions between the three major clusters (non-Khoisan, northwestern Kalahari and southeastern Kalahari) in Fig. 1b . This suggests historical gene flow; however, PCA does not constitute a formal test of admixture. We next created a filtered data set, excluding individuals who were outliers with respect to others from the same self-identified ethno-linguistic group ( Supplementary Table S2 , Supplementary Fig. S7 ). Formal tests for a history of mixture ('three-population tests' [26] ) confirmed many examples of population mixture ( Supplementary Table S3 ). Most populations are admixed between a non-Khoisan population and a population from either the northwestern Kalahari or the southeastern Kalahari cluster ( Supplementary Table S3 ). The one exception is the Naro, who are genetically admixed between northwestern and southeastern Kalahari populations, just as they are intermediate geographically ( Fig. 1a ). Several Khoisan populations which are at the extremes of Fig. 1b , -- the Ju|'hoan_North, Ju|'hoan_South, Hoan, Taa_North and Taa_East—do not show evidence of admixture by formal three-population tests; some of these also show no evidence of admixture in STRUCTURE-like analyses ( Supplementary Fig. S8 ). This is intriguing because if these populations were indeed unadmixed, they could be used as representatives of the ancestral northwestern and southeastern Kalahari populations. However, the three-population tests have limited power, and STRUCTURE-like methods may not be able to detect admixture if there is no unadmixed relative in the data set ( Supplementary Fig. S9 ). We therefore developed a novel test for admixture that takes advantage of the fact that if and only if population mixture occurred, we expect to detect linkage disequilibrium (LD)—non-random association of SNP genotypes—that is correlated to the allele frequency differences between the two ancestral populations [27] , [28] ( Supplementary Fig. S10 ). In all five populations, we observe that LD decays exponentially with genetic distance. This is evidence that all Khoisan populations in our study, even the most isolated, are admixed with non-Khoisan populations ( Fig. 2a ; Supplementary Figs S11, S12 ). 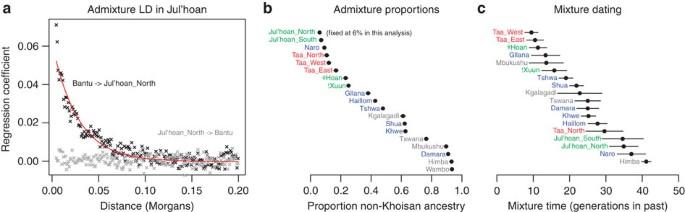Figure 2: All Khoisan populations are admixed. (a) Admixture linkage disequilibrium (LD) in the Ju|'hoan_North. For each pair of SNPs in the Ju|'hoan_North (black) or the Yoruba (grey), we estimate the LD and the product of the differences in allele frequency between the Ju|'hoan_North and the Yoruba. (We use the Yoruba as a proxy for the non-Khoisan, presumably Bantu-speaking ancestral population because there has been very little change in allele frequencies between Niger-Congo-speaking groups.) We then binned pairs of SNPs by the genetic distance between them. For each bin, we plot the regression coefficient (over SNP pairs in the bin) from regressing the level of LD on the product of the allele frequency differences. The rate at which this curve decays is informative about the date of admixture, whereas the amplitude of the curve is informative about the proportion of admixture (Supplementary Methods). In black is the curve if we assume the Ju|'hoan_North are admixed; in grey is the curve if we assume the Yoruba are admixed (which serves as a negative control). The red line is the exponential curve fitted to the black points. (b) Estimates of mixture proportions. We used the modifiedf4ratio19(Supplementary Methods) to estimate the fraction of non-Khoisan ancestry in each southern African population. (c) Estimates of mixture dates. We used the rate at which admixture LD decays to estimate dates of admixture for all southern African populations (Supplementary Methods). We plot the means, with ranges representing one standard error. Not shown are the Wambo, who have no detectable curve and hence may be unadmixed. The estimates of the mixture proportions and dates are also presented inSupplementary Table S4. Figure 2: All Khoisan populations are admixed. ( a ) Admixture linkage disequilibrium (LD) in the Ju|'hoan_North. For each pair of SNPs in the Ju|'hoan_North (black) or the Yoruba (grey), we estimate the LD and the product of the differences in allele frequency between the Ju|'hoan_North and the Yoruba. (We use the Yoruba as a proxy for the non-Khoisan, presumably Bantu-speaking ancestral population because there has been very little change in allele frequencies between Niger-Congo-speaking groups.) We then binned pairs of SNPs by the genetic distance between them. For each bin, we plot the regression coefficient (over SNP pairs in the bin) from regressing the level of LD on the product of the allele frequency differences. The rate at which this curve decays is informative about the date of admixture, whereas the amplitude of the curve is informative about the proportion of admixture ( Supplementary Methods ). In black is the curve if we assume the Ju|'hoan_North are admixed; in grey is the curve if we assume the Yoruba are admixed (which serves as a negative control). The red line is the exponential curve fitted to the black points. ( b ) Estimates of mixture proportions. We used the modified f 4 ratio [19] ( Supplementary Methods ) to estimate the fraction of non-Khoisan ancestry in each southern African population. ( c ) Estimates of mixture dates. We used the rate at which admixture LD decays to estimate dates of admixture for all southern African populations ( Supplementary Methods ). We plot the means, with ranges representing one standard error. Not shown are the Wambo, who have no detectable curve and hence may be unadmixed. The estimates of the mixture proportions and dates are also presented in Supplementary Table S4 . Full size image To estimate the proportion of admixture in the different Khoisan populations and to estimate when it occurred, we performed a quantitative analysis of the LD decay. Using population genetic theory presented in the Supplementary Methods , we show how the proportion of admixture can be derived from the amplitude of the exponential curve, that is, the point from which LD begins to decay. It has previously been shown that the time since admixture can be derived from the rate of LD decay [27] , [29] , [30] , and we also use this information below. The amplitude provides evidence of ∼ 6% non-Khoisan ancestry in the Ju|'hoan_North ( Fig. 2a , Supplementary Methods ). We then inferred the admixture proportions in the other southern Africans using a modified f 4 ratio estimate [19] that accounts for the admixture in the reference population ( Fig. 2b , Supplementary Table 4 , Supplementary Methods ). The estimated proportion of non-Khoisan ancestry in non-Bantu speakers ranges from 6% (Ju|'hoan_North) to around 90% (Damara; Fig. 2b ). We next estimated the time of admixture based on the extent of the LD. Ideally, we would like to infer a distribution of times to learn when the gene flow began and when it reached its peak [31] , but with current methods it is not possible to make robust statements about mixture events that are older than a dozen generations (because of errors in inference of local ancestry) [30] . Instead, we estimate a single date for the gene flow, which can be thought of as the weighted average of the admixture times [27] . We estimated this separately in each southern African population ( Fig. 2c ; Supplementary Table S4 , Supplementary Fig. S13 ). The earliest dates are around 40 generations ( ∼ 1,200 years) in the past, and the most recent dates are within the past few hundred years (though many of the populations with recent dates show evidence of additional gene flow before this; Supplementary Fig. S14 ). These dates are consistent with archeological evidence for the arrival of both East African pastoralists and agriculturalists (probably Bantu speakers) in southern Africa 2,000–1,200 years ago [32] , [33] , [34] , [35] . PCA suggests that the majority of admixture in the Khoisan is more closely related to the Yoruba (from West Africa, linguistically related to Bantu speakers) than to the Dinka (from northeastern Africa; Supplementary Fig. S5 ), although our data are consistent with additional East African ancestry in some Khoe speakers ( Supplementary Methods ). The two Khoisan groups split within the last 30,000 years To infer the date of population separation between the northwestern and southeastern Kalahari Khoisan, we developed a new methodology enabled by the design of the Human Origins array. The method is based on the rate at which Ju|'hoan-ascertained SNPs are observed to be monomorphic in the other populations. The excess of monomorphic SNPs beyond that expected due to genetic drift alone reflects new mutations that have arisen in the Ju|'hoan_North since the two populations split, and thus provides a measure of the time since the split ( Supplementary Methods , Supplementary Fig. S15 ). We verified that this approach can provide accurate estimates of population split dates by simulation ( Supplementary Figs S16, S17 ), and estimated that the split of the northwestern and southeastern Kalahari Khoisan occurred in the last 30,000 years ( Supplementary Figs S18, S19 ). However, this date is likely overestimated due to Bantu-related gene flow in these populations, and so should be treated as an upper bound ( Supplementary Fig. S17 ). A genetic link between southern and eastern Africa We examined two eastern African populations who speak languages with click consonants (Hadza and Sandawe) along with representative southern African populations using TreeMix [36] . This method fits a population graph—a generalization of a phylogenetic tree that incorporates the possibility of population mixture—to the allele frequency correlation patterns among a set of sampled populations. TreeMix infers that the Hadza are admixed between a Khoisan population (equally related to both the northwestern and southeastern Kalahari groups) and a population most closely related to the Dinka, with about 23±2% Khoisan-related ancestry ( Supplementary Fig. S20 ). The Sandawe show a similar signal, although weaker; TreeMix estimates that the Sandawe trace about 18±2% of their ancestry to admixture with a population related to the Khoisan ( Supplementary Fig. S21 ). TreeMix fits a single model to a large number of populations, and in principle, the finding of deep connections between southern and eastern Africans could be an artefact of modelling a complex history with a single admixture event. To explore the robustness of this finding, we used a four-population test [26] to determine whether the tree (Chimp, Ju|'hoan_North (Hadza, Dinka)) is a good fit to the genome-wide allele frequencies. This tree fails with a Z -score of −4.8 ( P =8×10 −7 ), indicating an excess of correlation in allele frequencies between the Ju|'hoan_North and Hadza. A consistent signal is seen in the Sandawe, although it is weaker ( Z -score of −2.1; P =0.018). Both the Hadza and the Sandawe show evidence of western Eurasian ancestry (perhaps reflecting gene flow from previously admixed neighbouring populations) [16] ; the weaker signal of relatedness between the Khoisan and the Sandawe may be due to a higher proportion of West Eurasian ancestry in the Sandawe ( Supplementary Fig. S22 ). These findings are consistent with the hypothesis that the Hadza and Sandawe harbour a proportion of their ancestry from a population related to southern Africans. Alternatively, more gene flow from an (as yet undiscovered) archaic human population into the ancestors of the Dinka than the Hadza (or Sandawe) could produce this signal. It has been suggested that the Mbuti and Biaka populations in central Africa may also be related to the Khoisan [16] , [17] ; whereas our analyses show that these populations do carry deep human lineages, they do not share the signal of relatedness to the Khoisan that we are focusing on here ( Supplementary Fig. S23 ). In sum, these results strongly suggest a genetic link between populations in southern and eastern Africa who speak non-Bantu languages with heavy use of click consonants. Model for the relationship of southern and eastern Africans We used TreeMix to build a unified model for the ancestral relationships between the Khoisan and eastern African populations, taking into account the confounding factor that all the populations harbour recent admixture. To do this, we extended TreeMix to subtract out the effect of gene flow from non-Khoisan populations ( Supplementary Methods ). This analysis provides strong evidence for a shared origin for the Khoisan-related genetic material in the Hadza and Sandawe. The Khoisan-related ancestry in the Hadza and Sandawe forms one clade, whereas the southern African Khoisan form a second clade consisting of the northwestern and southeastern Kalahari groups ( Fig. 3 ). 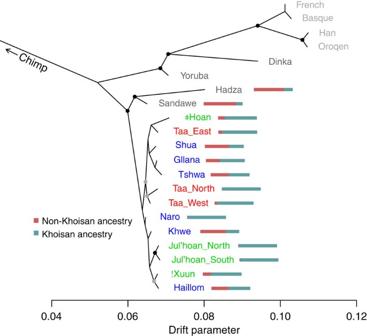Figure 3: Relationships among Khoisan and eastern Africans after removing non-Khoisan admixture. We extended TreeMix to build trees after subtracting out the effect of known admixture (Supplementary Methods) and then applied it to the Khoisan (excluding the Damara, who are genetically close to non-Khoisan). Populations are coloured according to their linguistic affiliation (Khoisan) or geographic location (dark grey=non-Khoisan African, light grey=Eurasian), and the chimpanzee was used as an out-group. The bar chart next to each population shows the estimated ancestry proportions for each population: blue is the proportion of Khoisan ancestry, and red is the proportion of non-Khoisan ancestry. Note that the actual source of these two ancestries may vary among populations. The proportions are not identical to those presented inFig. 2bbecause of small differences in how they are estimated. The black dots show splits supported by more than 95% of bootstrap replicates, and the grey dots those supported by more than 80% of bootstrap replicates. Figure 3: Relationships among Khoisan and eastern Africans after removing non-Khoisan admixture. We extended TreeMix to build trees after subtracting out the effect of known admixture ( Supplementary Methods ) and then applied it to the Khoisan (excluding the Damara, who are genetically close to non-Khoisan). Populations are coloured according to their linguistic affiliation (Khoisan) or geographic location (dark grey=non-Khoisan African, light grey=Eurasian), and the chimpanzee was used as an out-group. The bar chart next to each population shows the estimated ancestry proportions for each population: blue is the proportion of Khoisan ancestry, and red is the proportion of non-Khoisan ancestry. Note that the actual source of these two ancestries may vary among populations. The proportions are not identical to those presented in Fig. 2b because of small differences in how they are estimated. The black dots show splits supported by more than 95% of bootstrap replicates, and the grey dots those supported by more than 80% of bootstrap replicates. Full size image Our analysis of diverse southern and eastern African populations has documented deep structure in southern Africa that was previously unknown: a division between NW and SE Kalahari groups that arose within the past 30,000 years. We have also detected admixture in all Khoisan reflecting gene flow from Bantu-speaking agriculturalists and/or eastern African pastoralists within the past 1,200 years. Finally, we demonstrate an ancient link between the Khoisan and the Hadza and Sandawe in eastern Africa. This has implications for the geographic origin of modern humans, for which both eastern and southern Africa have been proposed [17] , [37] , [38] . Present-day populations in southern and eastern Africa are located on both sides of the deepest split of the tree ( Fig. 3 ), and thus from the perspective of phylogeography, our results are equally consistent with both of these locations as the origin of modern humans. Data The southern African samples included in this study were collected in various locations in Botswana and Namibia as part of a multidisciplinary project, after ethical clearance by the Review Board of the University of Leipzig and with prior permission of the Ministry of Youth, Sport and Culture of Botswana and the Ministry of Health and Social Services of Namibia. Approximately 2 ml of saliva were collected in tubes containing 2 ml of stabilizing buffer. Each sample was genotyped on the Affymetrix Human Origins array [19] and merged with additional samples [19] , [20] , [21] ( Supplementary Methods ). The SNPs on the Human Origins array are organized into panels of SNPs discovered in different individuals. Except where otherwise noted, we restrict ourselves to using the 150,425 autosomal SNPs discovered in a single Ju|'hoan_North (HGDP 'San') individual. The exceptions to this are all ROLLOFF analyses (for example, Fig. 2a,c ), where we used all 565,259 autosomal SNPs on the array. For analyses including the Hadza and Sandawe, some SNPs were removed because of genotyping or sequencing errors ( Supplementary Methods ); the corresponding number of Ju|'hoan-ascertained SNPs used when analysing these populations was 146,843. Analysis of population structure and mixture PCA was performed using smartpca [22] v9003. We tested for admixture using three- and four-population tests [19] . To estimate admixture dates, we used ROLLOFF v625 (ref. 27 ). To estimate the admixture proportion of the Ju|'hoan_North, we binned SNPs according to the genetic distance between them (with a bin size of 0.01 cM), and for each pair of SNPs we calculated the LD between them as well as the product of the allele frequency differences between the Ju|'hoan_North and the Yoruba. In each bin, we regressed the amount of LD against the product of allele frequency differences, and fit an exponential curve to the resulting regression coefficients. The intercept of the fitted exponential curve is expected to be f /(1- f ), where f is the mixture fraction (see Supplementary Methods for details). Estimating population divergence times To date the split between the NW and SE Kalahari groups, we developed a new method based on the fact that after the split of two populations, a given lineage from one of the populations accumulates mutations (that are not observed in the other population) at a clock-like rate that is proportional to years. Our method enables us to count these mutations, and convert this count to absolute time (see Supplementary Methods for details). Building population trees To build population trees in the presence of admixture, we modified the TreeMix model [36] . We first constructed a tree using unadmixed populations (Chimpanzee, Yoruba, Dinka, Europeans and East Asians) and then added admixed Khoisan populations to this tree using their estimated admixture proportions (see Supplementary Methods for details). How to cite this article: Pickrell, J. K. et al . The genetic prehistory of southern Africa. Nat. Commun. 3:1143 doi: 10.1038/ncomms2140 (2012).